Different thresholds of ZEB1 are required for Ras-mediated tumour initiation and metastasis Ras pathway mutation is frequent in carcinomas where it induces expression of the transcriptional repressor ZEB1. Although ZEB1 is classically linked to epithelial–mesenchymal transition and tumour metastasis, it has an emerging second role in generation of cancer-initiating cells. Here we show that Ras induction of ZEB1 is required for tumour initiation in a lung cancer model, and we link this function to repression Pten, whose loss is critical for emergence of cancer-initiating cells. These two roles for ZEB1 in tumour progression can be distinguished by their requirement for different levels of ZEB1. A lower threshold of ZEB1 is sufficient for cancer initiation, whereas further induction is necessary for tumour metastasis. Mutant Ras short circuits growth factor signalling by directly activating PI3K [1] , [2] , [3] . In an opposing manner, the tumour suppressor Pten inhibits PI3K function by dephosphorylation of its substrate phosphotidyl-inositol 3,4,5 triphosphate [4] . Ras pathway mutation, loss of PTEN and thus constitutive PI3K signalling are frequent in tumours and are hallmarks of lung and pancreatic cancer [2] , [3] , [4] . Although PTEN is frequently mutated in tumours, notably, it is not mutated in tumours with Ras mutations, but it is nevertheless repressed in these tumours [3] , [4] . It is unclear how Ras mutation might lead to repression of Pten, but such repression would allow a PI3K activator such as Ras to simultaneously block a PI3K inhibition pathway. Downregulation of PTEN appears crucial not only for maintenance of normal stem cells, but also for emergence of tumour-initiating cancer stem cells in tumours [3] , [4] . Thus, repression of Pten and constitutive PI3K activation appear to be critical for Ras-mediated tumour initiation. Another target of Ras pathway activation is the transcriptional repressor ZEB1 (refs 5 , 6 ). ZEB1 regulates epithelial–mesenchymal balance during development, but its expression is linked to cell proliferation through the Rb1 family and thus it is normally downregulated in most post-mitotic adult tissues [7] , [8] , [9] , [10] . Induction of ZEB1 in tumours drives epithelial–mesenchymal transition (EMT) that is thought to facilitate metastasis in later stage tumours, and accordingly its expression is correlated with poor prognosis [5] , [6] , [7] , [8] , [9] , [10] . Experimentally, overexpression and knockdown of ZEB1 in cancer cell lines has demonstrated its importance for tumour progression when these cells are transplanted into mice [5] , [6] . In addition, we demonstrated previously that induction of ZEB1 is required for viability and tumorigenity of Ras-transformed primary culture cells [8] , [11] . But, notably, tumours formed with these Ras-transformed primary cells were not metastatic, and the fact that ZEB1 was required for tumorigenicity implied that its induction is somehow critical for Ras-mediated tumour initiation. Interestingly, ZEB1 has been linked to induction of stem cell factors such as Bmi1 (reviewed in ref. 5 ), and recent studies demonstrate a critical role for induction of ZEB1 in generation of tumour-initiating cancer stem cells [12] , [13] . Taken together, such findings raise the possibility of a second, as yet uninvestigated, role for ZEB1 in Ras-mediated cancer initiation. Here we provide evidence that Ras induction of ZEB1 is required for tumour initiation is a Ras-mediated model of lung cancer. We demonstrate that ZEB1 directly represses Pten, and suggest that this Ras/ZEB1/Pten pathway allows Ras mutation to both activate PI3K and represses the PI3K pathway inhibitor Pten during tumour initiation, thereby explaining why there is no evidence of or requirement for Pten mutation in Ras-initiated tumours. We provide evidence that roles for ZEB1 in tumour initiation and EMT/metastasis can be separated based on their requirements for different levels of ZEB1: a low threshold of ZEB1 is sufficient for tumour initiation, whereas further induction is necessary for metastasis. Heterozygous mutation of ZEB1 blocks benign-to-malignant transition in Ras-initiated lung adenocarcinoma We examined a role for ZEB1 induction in cancer initiation in vivo . For these studies, we chose a model where activation of an oncogenic K-Ras allele by recombination in somatic cells triggers spontaneous lung cancer (K-Ras LA1 mice; ref. 14 ; Supplementary Fig. 1 ). In these mice, regions of atypical adenomatous hyperplasia (AAH) arise in bronchial airways, and this hyperplasia expands to initiate formation of subpleural benign adenomas ( Supplementary Fig. 1 ; Fig. 1a ). Small foci of adenocarcinoma then appear within these precancerous lesions as the first evidence of transition to malignancy ( Supplementary Fig. 1 ; Fig. 1b ). Multiple adenocarcinomas form in each lung, and these tumours then expand into surrounding airways ( Supplementary Fig. 1 ). But, notably, tumours in this model do not become metastatic, allowing a focus on tumour initiation. ZEB1 (−/−) mice are not viable, but ZEB1 (+/−) mice, which express approximately half the level of ZEB1, are viable [10] , [15] . Heterozygous mutation of ZEB1 is responsible for corneal dystrophy in mice and humans, and patients with this mutation also show increased risk for hernia, hydrocele and aneurysm [16] , [17] . Thus, a partial decrease in ZEB1 resulting from mutation of one allele is biologically significant, implying a narrow threshold linking ZEB1 expression to at least some functions. ZEB1 is not expressed in the developing or adult lung, and ZEB1 mutant mice do not display any obvious defect in lung development [10] , [15] . We crossed K-Ras LA1 mice into a ZEB1 (+/−) background and compared lung adenocarcinoma progression in ZEB1 (+/+) and ZEB1 (+/−) litter mates. Heterozygous mutation of ZEB1 did not significantly affect the number of adenomas, but remarkably, foci of adenocarcinoma failed to form, and none of the ZEB1 (+/−) mice developed lung cancer ( Fig. 1c ). These results provided surprising evidence that a threshold of ZEB1 induction is required for lung cancer initiation in these mice. To our knowledge, this is the first example of a heterozygous mutation serving to suppress cancer. 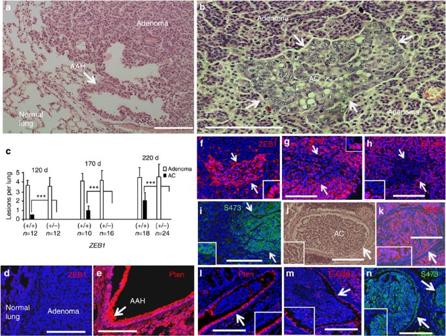Figure 1: ZEB1 is induced and Pten is repressed as precancerous adenomas transit to malignant adenocarcinoma (AC) in K-RasLA1mice, and heterozygous mutation ofZEB1blocks lung cancer initiation in these mice. (a) Sites of AAH originate in bronchial airways, and transit into numerous precancerous adenomas by 150 days of age. Haematoxylin and eosin (H&E) staining is shown. Also seeSupplementary Fig. 1. (b) H&E staining showing the appearance of foci of AC within an adenoma. Also seeSupplementary Fig. 1. (c) K-RasLA1mice were crossed withZEB1(+/−) mice and the effect ofZEB1heterozygous mutation on adenoma and AC formation was followed. s.d. are shown along with the significance calculated byT-test.n=number of mice. (d) Immunostaining showing that ZEB1 is not expressed in normal lung or in adenomas. (e) Pten is expressed in normal lung and AAH. (f–i) Immunostaining of sections adjacent to that inb. Arrows indicate the border of AC. (j) H&E section showing AC invasion into a large airway. The arrow indicates the border of the airway. (k–n) Immunostaining of sections adjacent to that inm. Scale bars, 100 μm. ***P<0.01 as calculated by T-test. Figure 1: ZEB1 is induced and Pten is repressed as precancerous adenomas transit to malignant adenocarcinoma (AC) in K-Ras LA1 mice, and heterozygous mutation of ZEB1 blocks lung cancer initiation in these mice. ( a ) Sites of AAH originate in bronchial airways, and transit into numerous precancerous adenomas by 150 days of age. Haematoxylin and eosin (H&E) staining is shown. Also see Supplementary Fig. 1 . ( b ) H&E staining showing the appearance of foci of AC within an adenoma. Also see Supplementary Fig. 1 . ( c ) K-Ras LA1 mice were crossed with ZEB1 (+/−) mice and the effect of ZEB1 heterozygous mutation on adenoma and AC formation was followed. s.d. are shown along with the significance calculated by T -test. n =number of mice. ( d ) Immunostaining showing that ZEB1 is not expressed in normal lung or in adenomas. ( e ) Pten is expressed in normal lung and AAH. ( f – i ) Immunostaining of sections adjacent to that in b . Arrows indicate the border of AC. ( j ) H&E section showing AC invasion into a large airway. The arrow indicates the border of the airway. ( k – n ) Immunostaining of sections adjacent to that in m . Scale bars, 100 μm. *** P <0.01 as calculated by T-test. Full size image Pten is repressed and Akt-S473 accumulates as ZEB1 is induced in foci of forming adenocarcinoma As opposed to ZEB1, Pten is repressed in Ras-driven tumours and even a partial decrease in Pten is sufficient to promote cancer initiation [4] , [18] . Pten is required for normal lung epithelial development, and deletion of Pten in the adult mouse lung epithelium leads to hyperplasia and adenocarcinoma [19] . Accordingly, Pten was expressed in normal lung, but ZEB1 was absent ( Fig. 1d,e ). Nor was ZEB1 evident in AAH or in benign adenomas, which continued to express Pten and the epithelial marker E-cadherin ( Fig. 1f–h ). Activation of mTorc2 by PI3K leads to mTor-catalyzed phosphorylation and activation of Akt on S473 (Akt-S473) [20] . Mutation of the mTorc2-specific component Rictor reverses the effects of Pten mutation in leukaemia [21] , demonstrating that the mTorc2/Akt-S473 pathway is an important downstream target of Pten (via PI3K) [4] . Consistent with Pten expression, Akt-S473 was absent in normal lung, AAH and adenomas ( Fig. 1i ). ZEB1 was induced, Pten and E-cadherin (a known target of ZEB1 repression [5] , [6] , [10] ) were repressed and Akt-S473 accumulated in foci of adenocarcinoma initiating within adenomas ( Fig. 1f–i ), and this pattern persisted as adenocarcinomas expanded into large airways ( Fig. 1j–n ). Induction of ZEB1 and repression of PTEN in Ras mutated human lung adenocarcinomas is a predictor of worse patient survival Next we examined ZEB1 and PTEN mRNA expressions in human lung adenocarcinoma microarrays ( Fig. 2a ). ZEB1 mRNA was higher in tumours with mutant K-Ras or an activating Ras pathway mutation in epidermal growth factor receptor (EGFR; n =25) than in tumours wild type for K-Ras and EGFR ( n =9), and PTEN mRNA levels inversely correlated with that of ZEB1 ( Fig. 2a,b ). Consistent with this diminished PTEN mRNA as a negative predictor of survival, a significant difference in patient survival was noted by simply dividing tumours into two groups based on PTEN mRNA levels ( Fig. 2c ). 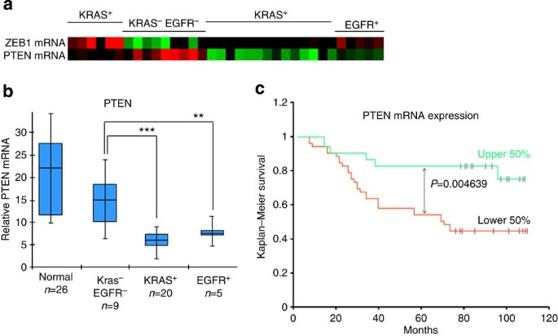Figure 2: ZEB1 and PTEN mRNA expression signatures predict survival in human lung adenocarcinoma. (a) Heat map showing relative expression of ZEB1 and PTEN mRNAs in human lung adenocarcinoma microarrays. K-Ras+and EGFR+indicate mutations, and K-Ras−and EGFR−indicate no mutations detected by sequencing. (b) Box plot showing expression of PTEN mRNA in human lung adenocarcinoma microarrays. The top of the box is the 75th percentile, whereas the bottom is the 25th percentile. The bar indicates the median and whiskers the highest and lowest values. ‘Normal’ indicates adjacent uninvolved lung tissue.n=the number of tumours. **P<0.05 and ***P<0.01 calculated byT-test. (c) Kaplan–Meier plot showing that PTEN mRNA expression predicts survival in human lung adenocarcinoma. Significance was calculated byT-test. Figure 2: ZEB1 and PTEN mRNA expression signatures predict survival in human lung adenocarcinoma. ( a ) Heat map showing relative expression of ZEB1 and PTEN mRNAs in human lung adenocarcinoma microarrays. K-Ras + and EGFR + indicate mutations, and K-Ras − and EGFR − indicate no mutations detected by sequencing. ( b ) Box plot showing expression of PTEN mRNA in human lung adenocarcinoma microarrays. The top of the box is the 75th percentile, whereas the bottom is the 25th percentile. The bar indicates the median and whiskers the highest and lowest values. ‘Normal’ indicates adjacent uninvolved lung tissue. n =the number of tumours. ** P <0.05 and *** P <0.01 calculated by T -test. ( c ) Kaplan–Meier plot showing that PTEN mRNA expression predicts survival in human lung adenocarcinoma. Significance was calculated by T -test. Full size image ZEB1 expression correlates with lack of PTEN and E-cadherin and accumulation of Akt-S473 in K-Ras mutated human lung adenocarcinomas To assess the pattern of protein expression within tumours, we immunostained representative human lung adenocarcinomas ( Fig. 3a–d ). By contrast to mouse models of lung adenocarcinoma where precancerous adenomas transit to malignant adenocarcinoma, adenomas are not evident in human lung adenocarcinomas. Instead, human adenocarcinoma in situ (AIS) with no invasive features is a localized, small precancerous lesion with growth restricted to a noninvasive lepidic pattern and an absence of papillary or micropapillary patterns or intra-alveolar tumour cells [22] . It is unclear whether AIS represents a precancerous transitional stage leading to human lung adenocarcinoma or whether it represents a terminal stage that never progresses to malignancy. Nevertheless, we observed that AIS expressed little ZEB1 and consistently PTEN was expressed ( Fig. 3c,d ). Thus, as in mouse adenoma, it appears that ZEB1 induction and PTEN loss are not evident in precancerous AIS lesions in human lung adenocarcinoma. Examining infiltrating lung adenocarcinomas, we found that ZEB1 expression did not overlap with that of PTEN or E-cadherin and it positively correlated with AKT-S473 ( Fig. 3a,b ). Consistent with the lower levels of ZEB1 mRNA and higher levels of PTEN mRNA seen in tumours lacking an activating Ras pathway mutation in K-Ras or EGFR ( Fig. 2a ), we found immunostaining of PTEN in these tumours, and ZEB1 was absent ( Fig. 3b ). This ZEB1-low, PTEN-high pattern was seen in nine tumours lacking a K-Ras or EGFR mutation. Taken together with the mouse studies above, these results suggest linkage between K-Ras pathway mutation, induction of ZEB1 and downregulation of PTEN. 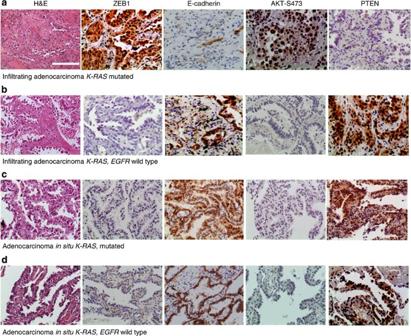Figure 3: ZEB1 and PTEN show distinct patterns of expression in human lung adenocarcinomas. Immunostaining of representative samples of human lung adenocarcinoma is shown. Tumour type and K-Ras and EGFR mutation status are shown below each panel. Scale bar, 100 μm. Figure 3: ZEB1 and PTEN show distinct patterns of expression in human lung adenocarcinomas. Immunostaining of representative samples of human lung adenocarcinoma is shown. Tumour type and K-Ras and EGFR mutation status are shown below each panel. Scale bar, 100 μm. Full size image A ZEB1-high, PTEN-low pattern is evident in the tumour stroma of K-Ras mutant lung adenocarcinomas We also examined the tumour stroma where ZEB1 has been shown previously to be expressed in some tumours [12] , [23] . Interestingly, we found that the same ZEB1-high, PTEN-low proliferating pattern seen in the K-Ras pathway mutant tumour cells was recapitulated in the tumour-associated stromal fibroblasts ( Supplementary Figs 2–5 ). By contrast, lung parenchyma near the tumour (but beyond the tumour margin) and fibroblasts in normal lung distal to the tumour showed an inverse ZEB1-low, PTEN-high non-proliferative pattern ( Supplementary Figs 2–5 ). Thus, a ZEB1 high, PTEN low proliferative signature is somehow transferred from tumour cells to adjacent fibroblasts. But how might a ZEB1-inducing K-Ras mutation in a tumour cell convey ZEB1 expression on an adjacent stromal cell? Although ZEB1 and proliferation marked fibroblasts in the tumour field, it is of note that these fibroblasts were not necessarily in direct contact with tumour cells, suggesting that cell–cell contact between fibroblasts and tumours cells is not required. Such proximity dependence then suggests release of an inducible factor from the tumours cells that acts on adjacent fibroblasts to induce ZEB1, repress PTEN and cause proliferation. Ras pathway mutation classically activates growth factors including transforming growth factor beta (TGF-β), which induces ZEB1 mRNA, represses Pten mRNA and causes cell proliferation ( Supplementary Fig. 6 ; refs 24 , 25 , 26 ). Thus, release of growth factors such as TGF-β from K-Ras mutant tumours might be sufficient for ZEB1 induction, PTEN repression and proliferation of tumour-associated fibroblasts. In support of this possibility, we found that serum-free conditioned media from primary culture of K-Ras-initiated mouse lung adenocarcinoma induced ZEB1 mRNA, repressed Pten mRNA and triggered proliferation of fibroblasts ( Supplementary Fig. 6 ). These results provide evidence that secreted factors from primary culture K-Ras-positive lung adenocarcinoma are sufficient for ‘activation’ of fibroblasts. Ras induction of ZEB1 is required for Pten repression and viability of mouse lung adenocarcinoma cells Next we evaluated the linkage between ZEB1 and Pten in primary cultures derived from K-Ras LA1 lung adenocarcinomas [27] . These 393P cells showed induction of ZEB1 mRNA, repression of Pten mRNA and accumulation of Akt-S473, and they formed tumours when transplanted back into mouse lungs, but these tumours were not metastatic ( Fig. 4a ; ref. 27 ). Knockdown of ZEB1 led to induction of Pten mRNA ( Fig. 4a ), and it triggered a block in proliferation and caused transition to multinucleated large, flat senescent cells ( Fig. 4b,c ), suggesting that the 393P cells had become addicted to ZEB1. Accordingly, the cells were no longer tumorigenic, demonstrating that ZEB1 induction is necessary for tumour initiation. If ZEB1 was further overexpressed (393P ZEB1), the cells then gave rise to highly metastatic lung tumours [27] , and knockdown of ZEB1 in these cells likewise caused loss of proliferation and viability ( Fig. 4c,d ). Consistent with repression of Pten mRNA, 393P cells showed constitutive Akt-S473, which persisted when ZEB1 was overexpressed in the cells ( Fig. 4e,f ). In addition, Akt-S473 was lost when ZEB1 was knocked down and Pten mRNA was induced ( Fig. 4g,h ). Taken together, these results link ZEB1 induction in 393P cells to Pten repression, accumulation of Akt-S473 and tumour initiation. However, a higher level of ZEB1 is required for transition to metastasis, where the elevated ZEB1 appears required to activate a pathway beyond Pten/Akt-S473. 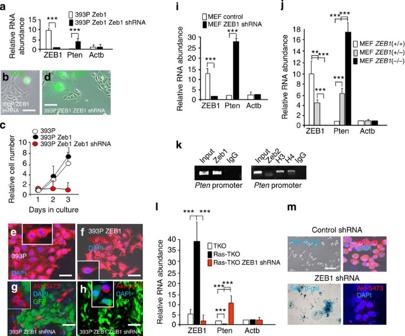Figure 4: Ras induction of ZEB1 represses Pten, and these cells become addicted to ZEB1. (a) Lentiviral shRNA knockdown of ZEB1 in 393P cells led to induction of Pten mRNA. Real-time PCR is shown. (b) Knockdown of ZEB1 in 393P cells leads to large, flat senescent cells. (c) ZEB1-knockdown 393P cells fail to proliferate. (d) Knockdown of ZEB1 in 393P ZEB1 cells also leads to large, flat senescent cells. (e,f) Immunostaining of Akt-S473 in 393P and 393P ZEB1 (forced overexpression of ZEB1). Note that Akt-S473 is not evident in normal lung or in adenomas. (g,h) Knockdown of ZEB1 with lentivirus shRNA eliminated Akt-S473. GFP is expressed from the lentivirus. (i) Real-time PCR showing Pten mRNA induction with lentiviral shRNA knockdown of ZEB1 in MEFs. Multiple shRNA sequences were used for knockdowns with similar results (see Methods), and the level of ZEB1 protein and RNA following knockdown was shown previously13. (j)ZEB1mutation leads to a gene dosage-dependent induction of Pten mRNA. Real-time PCR is shown. (k) ChIP assays showing binding of ZEB1 to thePtenpromoter. IgG indicates control antisera, and H3 and H4 are histone controls. (l) Real-time PCR showing Ras induction of ZEB1 mRNA and repression of Pten mRNA inRb1family triple-knockout MEFs (Ras-TKO). Lentiviral shRNA was then used to knockdown ZEB1 in the Ras-TKO MEFs as described13. (m) Knockdown of ZEB1 led to loss of Akt-S473 and senescence of Ras-TKO MEFs. Senescence was assessed by staining for senescent β-galactosidase (Sen β-Gal)10. Scale bars, 20 μM. s.d. are shown and ***P<0.01 and **P<0.5 byT-test. All results are representative of at least three independent experiments. Figure 4: Ras induction of ZEB1 represses Pten, and these cells become addicted to ZEB1. ( a ) Lentiviral shRNA knockdown of ZEB1 in 393P cells led to induction of Pten mRNA. Real-time PCR is shown. ( b ) Knockdown of ZEB1 in 393P cells leads to large, flat senescent cells. ( c ) ZEB1-knockdown 393P cells fail to proliferate. ( d ) Knockdown of ZEB1 in 393P ZEB1 cells also leads to large, flat senescent cells. ( e , f ) Immunostaining of Akt-S473 in 393P and 393P ZEB1 (forced overexpression of ZEB1). Note that Akt-S473 is not evident in normal lung or in adenomas. ( g , h ) Knockdown of ZEB1 with lentivirus shRNA eliminated Akt-S473. GFP is expressed from the lentivirus. ( i ) Real-time PCR showing Pten mRNA induction with lentiviral shRNA knockdown of ZEB1 in MEFs. Multiple shRNA sequences were used for knockdowns with similar results (see Methods), and the level of ZEB1 protein and RNA following knockdown was shown previously [13] . ( j ) ZEB1 mutation leads to a gene dosage-dependent induction of Pten mRNA. Real-time PCR is shown. ( k ) ChIP assays showing binding of ZEB1 to the Pten promoter. IgG indicates control antisera, and H3 and H4 are histone controls. ( l ) Real-time PCR showing Ras induction of ZEB1 mRNA and repression of Pten mRNA in Rb1 family triple-knockout MEFs (Ras-TKO). Lentiviral shRNA was then used to knockdown ZEB1 in the Ras-TKO MEFs as described [13] . ( m ) Knockdown of ZEB1 led to loss of Akt-S473 and senescence of Ras-TKO MEFs. Senescence was assessed by staining for senescent β-galactosidase (Sen β-Gal) [10] . Scale bars, 20 μM. s.d. are shown and *** P <0.01 and ** P <0.5 by T -test. All results are representative of at least three independent experiments. Full size image ZEB1 directly represses Pten K-Ras mutation also drives sarcoma initiation [28] where ZEB1 is induced and Pten is likewise downregulated, as opposed to mutated [28] , [29] , [30] , [31] , [32] . In addition, as noted above, a ZEB1 high/PTEN low pattern also marks fibroblasts in the stroma of K-Ras mutant tumours, and such loss of Pten in the tumour stroma has been shown to be important for tumour progression [33] . Together, these findings provide evidence of important links between K-Ras mutation, ZEB1 induction and Pten repression in mesenchymal cells. We therefore initiated studies on a potential Ras-ZEB1-Pten pathway in primary cultures of mouse fibroblasts. Heterozygous mutation of ZEB1 (ref. 10 ) was sufficient for induction of Pten mRNA, and short hairpin RNA (shRNA) knockdown of ZEB1 likewise led to induction of Pten mRNA in these cells ( Fig. 4i,j ). Chromatin immunoprecipitation (ChIP) assays showed ZEB1 bound to the Pten promoter in vivo ( Fig. 4k ), suggesting that it is directly repressing Pten . As a control, the ZEB family member, ZEB2, did not bind the Pten promoter ( Fig. 4k ). We conclude that the ZEB1-Pten pathway observed in vivo is evident in both adenocarcinoma cells and fibroblasts in culture, and this pathway is driven by ZEB1 repression of Pten. Interplay between the Rb1 pathway and Ras mutation in induction of ZEB1 We wanted to model the role for Ras in the ZEB1, Pten pathway in primary cells. However, introduction of mutant Ras into wild-type primary cells leads to tumour-suppressing oncogene-induced senescence mediated by activation of the Rb1 family of cell cycle inhibitors [34] . Accordingly, the Rb1 family represents a barrier to the development of lung adenocarcinoma in Ras LA1 mice [35] . Therefore, Rb1 is either mutated (rarely, primarily retinoblastoma and small cell lung cancer) or inactivated by deregulated cyclin-dependent kinase hyperphosphorylation (in most other tumours) in cancer [36] . Mutation of the Rb1 family then provides a permissive environment for Ras mutation, and introduction of mutant Ras into primary fibroblasts lacking Rb1 family members is sufficient for oncogenic transformation [11] , [37] . Rb1 represses ZEB1, and this repression is dominant over induction by Ras [8] , [38] . Thus, mutation or inactivation of the Rb1 family, a hallmark of tumours, is also required for Ras induction of ZEB1, and in breast cancer Rb1 hyperphosphorylation coincides with ZEB1 induction [39] . Accordingly, we found that mutant Ras induced ZEB1 mRNA in primary cells when the Rb1 family was mutated, and these cells also showed repression of Pten mRNA and constitutive Akt-S473 ( Fig. 4l,m ). As in primary cells from mouse K-Ras-driven adenocarcinoma, knockdown of ZEB1 reversed this repression of Pten mRNA and it eliminated Akt-S473 in the fibroblasts ( Fig. 4l,m ). These findings demonstrate that Ras induction of ZEB1 is necessary for repression of Pten and accumulation of Akt-S473. As with the primary cultures derived from K-Ras-initiated lung adenocarcinoma, knockdown of ZEB1 in these Ras-transformed primary fibroblasts led to senescence and loss of cell viability ( Fig. 4m ), demonstrating that the cells are addicted to elevated ZEB1. It is then of note that introduction of mutant Ras into these Rb1 family null primary fibroblasts was sufficient for tumorigenesis when the cells were transplanted into nude mice [8] , [11] , and knockdown of ZEB1 in these cells to reverse its induction by Ras prevented tumour initiation [8] , [11] . Thus, ZEB1 induction is required for the tumour-initiating capacity of Ras in these cells. It was demonstrated previously that, as would be expected, knockdown of Akt eliminated Akt-S473 in these Ras-transformed fibroblasts [11] . However, as with the knockdown of ZEB1, these Akt-knockdown cells lost viability [11] . By contrast, knockdown of Akt in parent wild-type mouse embryo fibroblasts (MEFs) did not cause such a loss in viability [11] . It is then likely that ZEB1 addiction in the Ras-transformed cells reflects their dependence on constitutive Akt-S473. Delivery of lentiviral ZEB1 shRNA to the lung blocks progression of benign adenomas to adenocarcinoma Above we demonstrated that heterozygous ZEB1 mutation prevents transition of precancerous lesions to lung cancer in K-Ras LA1 mice. Because of the potential therapeutic implications of these findings, we wondered whether a partial reduction in ZEB1 expression after the onset of adenomas might still prevent transition to lung cancer. Adenomas initiate at 2 weeks of age in K-Ras LA1 mice [14] . Beginning at 1 month of age, lentivirus-expressing ZEB1 shRNA [13] or a control scrambled sequence was delivered intratracheally to K-Ras LA1 mice every 2 weeks until 3 months of age ( Fig. 5a–d ). These lentiviruses express green fluorescent protein (GFP), allowing us to follow viral infection. We found that infection occurred efficiently in most distal bronchial epithelial cells where AAH initiates, and a high percentage of alveolar cells were also infected ( Fig. 5b ). Even though viral delivery was stopped at 3 months of age, this pattern of GFP expression persisted in control mice and extended to form adenomas and adenocarcinomas. All control K-Ras LA1 mice died by 320 days of age ( Fig. 1b ), a pattern similar to untreated mice and to previous reports of survival [14] . We assessed lungs of these mice as they died. We did not observe an effect of control lentivirus on the number of adenomas or adenocarcinomas ( Fig. 5a ), and adenomas and adenocarcinomas that formed expressed GFP demonstrating that they were arising from infected cells. Only one of the ZEB1 shRNA lentivirus-treated mice died by 320 days of age, and this mouse showed severe pneumonia, perhaps associated with tracheal delivery of the virus ( Fig. 5a ). ZEB1 shRNA lentivirus-treated mice showed a similar pattern of GFP expression as a marker of infection. Histological assessment of these treated mice showed that they had developed adenomas ( Fig. 5a–d ), which expressed GFP, suggesting that they arose from cells infected by ZEB1 shRNA lentivirus. In addition, we observed a total of three adenocarcinomas in the lungs of these mice, but none of these adenocarcinomas expressed GFP ( Fig. 5a–d ), indicating that they arose from uninfected cells. 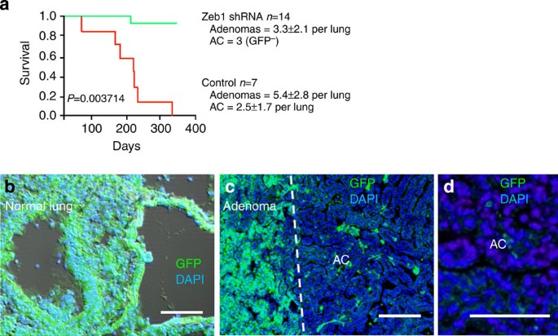Figure 5: Delivery of lentiviral ZEB1 shRNA to the lung inhibits lung adenocarcinoma (AC) and prolongs survival of K-RasLA1mice. (a) A Kaplan–Meier plot is shown. ‘Control’ indicates a virus with a scrambled shRNA sequence. (b–d) Frozen sections of the three ACs seen following treatment with lentiviral ZEB1 shRNA (a) were stained with DAPI and evaluated for GFP expression as a marker of lentiviral infection. Note that normal lung was efficiently infected, and adenomas also expressed GFP, but the three ACs that formed failed to express GFP, demonstrating that they all arose from uninfected cells in the lungs. One of these ACs is shown here. Scale bars, 100 μm.n=number of mice. Figure 5: Delivery of lentiviral ZEB1 shRNA to the lung inhibits lung adenocarcinoma (AC) and prolongs survival of K-Ras LA1 mice. ( a ) A Kaplan–Meier plot is shown. ‘Control’ indicates a virus with a scrambled shRNA sequence. ( b – d ) Frozen sections of the three ACs seen following treatment with lentiviral ZEB1 shRNA ( a ) were stained with DAPI and evaluated for GFP expression as a marker of lentiviral infection. Note that normal lung was efficiently infected, and adenomas also expressed GFP, but the three ACs that formed failed to express GFP, demonstrating that they all arose from uninfected cells in the lungs. One of these ACs is shown here. Scale bars, 100 μm. n =number of mice. Full size image Here we demonstrate that Ras induction of ZEB1 causes repression of Pten . This induction of ZEB1 allows a single Ras mutation to constitutively activate PI3K, while also eliminating repression of PI3K function by Pten, thus explaining the low frequency of Pten mutations in tumours initiated by mutant Ras. ZEB1 can act as a transcriptional activator as well as a repressor, depending on promoter context [5] , [6] . We found previously that ZEB1 can induce expression of mTor [11] , raising the possibility that beyond causing loss of Pten to activate mTorc2 (via PI3K-dependent phosphorylation) it may also facilitate assembly of mTorc2 by inducing expression of its catalytic subunit. Pten downregulation drives the early precancerous acinar-to-ductal metaplasia leading to panIN in progression to pancreatic cancer [40] . Pten downregulation is also required for cancer stem cell generation and maintenance [3] , [4] , [41] , and induction of ZEB1 can drive generation of cells with properties of cancer stem cells [5] , [12] , [13] , [40] . We then propose that the role for ZEB1 in cancer initiation and cancer stem cell generation is linked to its repression of Pten. We found that factors secreted from lung adenocarcinoma cells can induce ZEB1 mRNA, repress Pten mRNA and trigger fibroblast proliferation, suggesting a mechanism through which this pattern can be transferred from tumour cells to adjacent fibroblasts. Mutation of Pten in the tumour stroma is sufficient to facilitate breast cancer initiation [33] , [42] , implying an important function for downregulation of Pten in tumour-associated fibroblasts. Indeed, it has been demonstrated recently that Pten can be secreted and taken up by adjacent cells [43] , raising the possibility that elimination of Pten in fibroblasts is necessary to remove a secondary source of secreted Pten that would otherwise be taken up by adjacent tumour cells. K-Ras mutation also drives sarcoma initiation [28] where ZEB1 is induced and Pten is likewise downregulated as opposed to mutated [28] , [29] , [30] , [31] , [32] . Thus, the ZEB1, PTEN pathway can be induced by K-Ras in mesenchymal cells in the absence of adjacent carcinoma cells. We demonstrate this in cell culture as well. Consistent with the importance of ZEB1 induction in sarcoma, knockdown of ZEB1 blocked Ras-induced transition of primary fibroblasts to sarcoma [11] . These results raise the question as to whether a common mechanism might account for K-Ras induction of ZEB1 in tumours and induction of ZEB1 in adjacent fibroblasts. Previous studies of a human tumour cell line suggested that Ras activation of Erk2 was mediating induction of ZEB1 (ref. 7 ). However, in primary cells, we found that Erk activation was not required for Ras induction of ZEB1 (ref. 44 ). Thus, the mechanism through which Ras induces ZEB1 is still unresolved. Because ZEB1 expression is dependent on growth factors including TGF-β, which are induced by Ras, one hypothesis is that Ras mutation is inducing ZEB1 expression via these secreted growth factors, allowing Ras mutation in tumour cells to cause the same induction of ZEB1 and repression of Pten in adjacent fibroblasts. Repression of Pten has been linked to other EMT-associated factors including TGF-β and snail transcription factor [24] , [45] , [46] . These findings rise the possibility that ZEB1 upregulation is one of the mechanisms through which EMT can be linked to Pten repression. However, it has been demonstrated that Snail induces ZEB1 (ref. 47 ), implying a possible link between Snail and ZEB1 in Pten repression, at least under some conditions. Although various mechanisms, including induction of microRNAs (miRNAs) such as mir21 that target Pten mRNA, have been put forth as a mechanism of Pten repression by TGF-β [24] , [45] , we wondered whether induction of ZEB1 might also be mediating TGF-β repression of Pten. Therefore, we tested the effect of TGF-β on ZEB1 (−/−) MEFs. TGF-β failed to repress Pten mRNA in the ZEB1-null cells, and it failed to induce proliferation of the cells ( Supplementary Fig. 6 ). As a positive control for the TGF-β pathway in ZEB1 (−/−) fibroblasts, we demonstrated previously Tgf-β-induced target genes including Pai1 in these cells [10] . These results provide evidence that TGF-β repression of Pten is mediated through induction of ZEB1. Pten mutation has little effect on hematopoietic stem cell differentiation before adulthood, but Pten becomes a critical tumour suppressor of leukaemia in adults [21] . Because of the linkage between ZEB1 and Pten we show here, it is of note that ZEB1 expression is closely linked to cell proliferation during development, and it is therefore downregulated in most post-mitotic adult cells [10] . ZEB1 then becomes of consequence in adults when it is induced on oncogenic transformation (for example, by K-Ras). We suggest that this induction of ZEB1 serves initially to downregulate Pten, thereby conveying stemness features characteristic of cancer stem cells. Heterozygous mutation of Pten is sufficient to promote cancer initiation [3] , [4] , demonstrating a narrow window of functional expression. Correspondingly, heterozygous mutation of the Pten repressor, ZEB1 , is sufficient to increase Pten expression and prevent malignant transition in K-Ras-driven mouse lung cancer. This functional significance of partial repression of ZEB1 expression points to its potential as an important therapeutic target. It is of note that K-Ras mutation alone in the mouse lung leads to precancerous adenomas that transit to malignant adenocarcinoma, but these tumours do not become metastatic. However, as noted above, overexpression of ZEB1 in primary cultures of K-Ras-initiated mouse lung adenocarcinoma caused transition to metastatic disease, implying that a higher threshold of ZEB1 is sufficient to drive transition to metastatic disease, as suggested previously [27] , [48] . In this regard it is of note that combining K-Ras mutation with tumour-suppressor mutations in p53 or Ink4 leads to metastatic lung adenocarcinoma (reviewed in ref. 49 ). Might these tumour-suppressor mutations somehow lead to further induction of ZEB1 (beyond K-Ras alone) in transition to metastasis? p53 induces miRNAs including miR200 that normally target ZEB1, and with p53 mutation, these miRNAs are downregulated allowing for post-transcriptional ZEB1 induction [50] , [51] . Ink4 encodes the p53 regulatory factor Arf, and loss of Arf leads in turn to loss of p53 (refs 34 , 36 ). Further, Ink4 also encodes the cyclin-dependent kinase (cdk) inhibitor p16, which blocks activity of cyclin D-cdk4/6 (ref. 36 ). With loss of p16 inhibition on Ink4 mutation, constitutively active cyclin D-cdk4/6 hyperphosphorylates and fully inactivates Rb1. ZEB1 transcription is directly repressed by Rb1 (refs 8 , 38 ), thus loss of p53 and full inactivation of Rb1 resulting from these tumour-suppressor mutations might induce ZEB1 both transcriptionally and post-transcriptionally beyond the level seen with K-Ras mutation alone to a threshold sufficient for metastasis. Cell culture Rb1 family mutant MEFs and control wild-type MEFs were kind gifts from G. Leone and T. Jacks [37] . Cells derived from four separate embryos were used with similar results. 393P and 393P ZEB1 mouse lung adenocarcinoma cells were a kind gift from J. Kurie [27] . MEFs and ZEB1 mutant MEFs were isolated as described [10] . Cells were cultured in DMEM with 10% heat-inactivated fetal bovine serum [13] . Ras-TKO MEFs were created by infection with a V12 Ras retrovirus as described [44] . The resulting cells were characterized with regard to Ras expression by western blot, and Ras activity was carried out by using the EZ-Detect Ras Activation Kit (Pierce Biotechnology, Rockford, IL) GST fusion protein containing the Ras-binding domain of Raf [44] . RNA extraction and real-time PCR RNA was extracted using TRIzol (Invitrogen, Carlsbad, CA). Complementary DNA was synthesized using the Invitrogen RT Kit according to the manufacturer’s protocol (Invitrogen). SYBR Green real-time quantitative PCR was performed using the Mx3000P Real-Time PCR System (Stratagene, Cedar Creek, TX) according to the manufacturer’s instructions. PCR primers are shown in Supplementary Table 1 . Three independent samples, each in triplicate, were analysed for each real-time PCR condition, and products were analysed for size by agarose gel. ChIP assays were based on the Upstate Biotechnology protocol ( http://www.millipore.com/userguides/tech1/789mrn ) using formaldehyde to crosslink genomic DNA. Polyclonal antiserum for ZEB1 (ref. 10 ), histones H3 and H4 (Santa Cruz Biotechnology, Santa Cruz, CA) were used for immunoprecipitation. Equal amounts of anti-IgG or preimmune serum were used as negative controls, whereas histone H4 served as a positive control. ChIP PCR reactions were similar to those described above for real-time PCR. ChIP PCR primers are shown in Supplementary Table 2 . Three independent samples, each in triplicate, were analysed for each real-time PCR condition. Knockdown of ZEB1 We have described lentiviral shRNA knockdown of ZEB1 protein and mRNA previously [11] , [13] . To generate a lentivirus expressing ZEB1 shRNA, a primer containing a ZEB1 shRNA sequence (5′-CTGTCTAGACAAAAAAAGACAACGTGAAAGACAATCTCTTGAATTGTCAAACACGTTGTCTTGGGGATCTGTGGTCTCATACA-3′) was used with a T3 primer to amplify a 500-base-pair fragment containing the H1 promoter using the pSuper vector as a template. The resulting PCR product was digested with SpeI and XbaI and cloned back into the lentiviral vector digested with NheI. We first cloned the shRNA sequence into a CMV-GFP lentiviral vector, where its expression was driven by the mouse U6 promoter. Briefly, the shRNA construct was generated by synthesizing an 83-mer oligonucleotide containing: (i) a 19-nucleotide sense strand and a 19-nucleotide antisense strand, separated by a nine-nucleotide loop (5′-TTCAAGAGA-3′); (ii) a stretch of five adenines as a template for the Pol III promoter termination signal; (iii) 21 nucleotides complementary to the 3′ end of the Pol III U6 promoter; and (iv) a 5′ end containing a unique XbaI restriction site. The long oligonucleotide was used, together with a sp6 oligonucleotide (5′-ATTTAGGTGACACTATAGAAT-3′), to PCR amplify a fragment containing the entire U6 promoter plus shRNA sequences; the resultant product was digested with XbaI and SpeI ligated into the NheI of the lentivirus vector, and the insert was sequenced to ensure that no errors occurred during the PCR or cloning steps. Lentiviral particles were produced by a four-plasmid transfection system. Briefly, 293T cells were transfected with the lentiviral vector and packaging plasmids, and the supernatants, containing recombinant pseudolentiviral particles, were collected from culture dishes on the second and third days after transfection. TKO MEFs and Ras-TKO MEFs were transduced with these lentiviral particles expressing shRNAs targeting ZEB1. Beyond this original shRNA, we used five additional shRNA lentiviruses with different ZEB1 shRNA sequences from Open Biosystems for knockdowns with similar effects. Lentivirus with a scrambled shRNA sequence 5′-CAACAAGATGAAGAGCACCAATCTCTTGAATTGGTGCTCTTCATCTTGTTG-3′ was used as a control—this control sequence was blasted against all mouse RNA sequences to insure that it did not target an mRNA [13] . Immunostaining Immunostaining was performed as described previously [13] . Cells were washed with PBS, fixed with 4% formaldehyde for 10 min and then washed again with PBS. The cells were then treated with methanol at −20 °C for 10 min and blocked with 4% goat serum at room temperature for 1 h. The cells were incubated with primary antibody overnight at 4 °C. The next day, cells were washed with PBS followed by incubation with secondary antibody (Alexa Fluor goat anti-rabbit IgG, Invitrogen, Carlsbad, CA) for 1 h at room temperature. Images were captured with a Zeiss confocal microscope. Antibodies are described in Supplementary Table 3 . K-Ras LA1 mice Housing and handling of all mice were in accordance with procedures approved by the University of Louisville Institutional Animal Care and Use Committee (IACUC). K-ras LA1 mice [14] in a C57BL/6 background were obtained from Jackson Laboratory. These mice were crossed with ZEB1 (+/−) mice also in a C57BL/6 background [10] to yield K-Ras LA1 , ZEB1 (+/+) and K-Ras LA1 , ZEB1 (+/−) mice. Lungs were obtained for histological analysis of tumours at the indicated ages. PCR genotyping was as described previously [10] . Tumour pathology was evaluated independently by two experienced pathologists (A.B.J. and M.C.). For lentiviral ZEB1 shRNA or control shRNA treatment, K-Ras LA1 mice at 1 month of age were anaesthetized by IP injection of a combination of ketamine (100 mg kg −1 ) and xylazine (10 mg kg −1 ). The anaesthetized mouse was placed on a warm platform in a biosafety hood. The mouth was opened by gently pulling the upper two front teeth, the tongue was extended by the forceps and an Excel Saflet IV catheter was placed in the trachea. A total of 50 μl of DMEM cell supernatant with a viral titre of ~1 × 10 9 lentiviral particles was slowly delivered into the lung. The treated mice were then housed in a biosafety room and closely monitored daily in accordance with protocols approved by the Institutional Animal Care and Use Committee. This tracheal viral delivery was repeated every 2 weeks until the animals were 3 months of age. At this age, viral delivery was stopped. Human lung adenocarcinoma microarray and tissue analysis Microarray data for human lung adenocarcinomas sequenced for mutations in K-RAS and EGFR and patient-matched control lung tissue were obtained from the NCBI database (GSE_11969) [52] . Data were corrected for background and normalized to median fluorescence and GAPDH expression. Box plots were performed as described [18] . Formalin-fixed, paraffin-embedded sections of human lung adenocarcinomas were obtained from IDIBAPS’ Tumour Bank and their use was approved by the ethics committee. How to cite this article: Liu, Y. et al. Different thresholds of ZEB1 are required for Ras-mediated tumour initiation and metastasis. Nat. Commun. 5:5660 doi: 10.1038/ncomms6660 (2014).